Extraordinary momentum and spin in evanescent waves Momentum and spin represent fundamental dynamic properties of quantum particles and fields. In particular, propagating optical waves (photons) carry momentum and longitudinal spin determined by the wave vector and circular polarization, respectively. Here we show that exactly the opposite can be the case for evanescent optical waves. A single evanescent wave possesses a spin component, which is independent of the polarization and is orthogonal to the wave vector. Furthermore, such a wave carries a momentum component, which is determined by the circular polarization and is also orthogonal to the wave vector. We show that these extraordinary properties reveal a fundamental Belinfante’s spin momentum, known in field theory and unobservable in propagating fields. We demonstrate that the transverse momentum and spin push and twist a probe Mie particle in an evanescent field. This allows the observation of ‘impossible’ properties of light and of a fundamental field-theory quantity, which was previously considered as ‘virtual’. It has been known for more than a century, since the seminal works by J.H. Poynting [1] , that light carries momentum and angular momentum (AM) [2] , [3] . These are the main dynamical properties of electromagnetic waves, which are also preserved in the quantum-mechanical picture of photons [4] . Optical momentum and AM play a crucial role in various light-matter interactions [5] , [6] , [7] , including laser cooling [8] , [9] , [10] , optical manipulation of atoms or small particles [8] , [9] , [10] , [11] , [12] , [13] , and in optomechanical systems [14] . The simplest example of an optical field carrying momentum and spin AM is an elliptically polarized plane wave. Assuming free space propagation along the z axis, the complex electric field of such wave can be written as Here A is the wave amplitude, and are unit vectors of the corresponding axes, the complex number m determines the polarization state with being the helicity (ellipticity of polarization), k = ω / c is the wave number, and throughout the paper we imply monochromatic fields with omitted exp(− iωt ) factor. The momentum and spin AM in wave (1) can be characterized by the corresponding spatial densities where w = γω | A | 2 is the energy density, and we use Gaussian units with γ =(8 πω ) −1 . In agreement with the quantum-mechanical picture of photons [4] , the momentum p is determined by the wave vector and is independent of polarization. At the same time, the spin s is proportional to the polarization helicity σ and is also collinear with the wave vector. The optical momentum and spin densities can be measured experimentally by placing a small absorbing particle in the field and observing its linear and spinning motion [15] , [16] , [17] , [18] , [19] . Naturally, the radiation force and torque (with respect to the particle’s centre) quantify the momentum and AM transfer to the particle and are proportional to the densities (2) in the plane wave (1): F ∝ p and T ∝ s (refs 19 , 20 , 21 , 22 , 23 , 24 , 25 ), Fig. 1 . 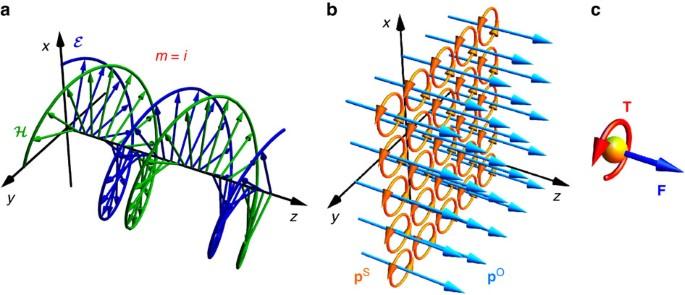Figure 1: Momentum and spin in a circularly-polarized propagating plane wave. The complex wave electric field is given by equation (1) withm=i, that isσ=1. (a) Instantaneous electric and magnetic fields, (r,t)=Re[E(r)e−iωt] and (r,t)=Re[H(r)e−iωt], form helical distributions (see alsoSupplementary Note 2andSupplementary Fig. 1). As the wave propagates along thezaxis, the fields rotate in the transverse (x,y) plane. This rotation generates the spin AM density, which is represented in (b) by multiple loops of the (zero-net) spin-momentumpS=∇×s/2 in the transverse plane. At the same time, the wave propagation produces the canonical (orbital) momentum density. (c) Orbital momentum and spin AM are locally transferred to a probe particle, thereby exerting a radiation forceF∝pOand torqueT∝son it, equation (6). Figure 1: Momentum and spin in a circularly-polarized propagating plane wave. The complex wave electric field is given by equation (1) with m=i , that is σ =1. ( a ) Instantaneous electric and magnetic fields, ( r , t )=Re[ E ( r ) e − i ω t ] and ( r , t )=Re[ H ( r ) e − i ω t ], form helical distributions (see also Supplementary Note 2 and Supplementary Fig. 1 ). As the wave propagates along the z axis, the fields rotate in the transverse ( x , y ) plane. This rotation generates the spin AM density , which is represented in ( b ) by multiple loops of the (zero-net) spin-momentum p S = ∇ × s /2 in the transverse plane. At the same time, the wave propagation produces the canonical (orbital) momentum density . ( c ) Orbital momentum and spin AM are locally transferred to a probe particle, thereby exerting a radiation force F ∝ p O and torque T ∝ s on it, equation (6). Full size image The above picture is simple and intuitively clear in the plane-wave case, but complex, spatially-inhomogeneous fields require a more careful approach. Below we show that one of the simplest examples of an inhomogeneous field—a single evanescent wave—exhibits extraordinary momentum and spin properties, which are in sharp contrast to what is known about photons, optical momentum and spin. Momentum and spin densities from field theory The momentum density p ( r ) of a quantum or classical wave field appears in the energy-momentum tensor within the corresponding field theory [26] , where momentum density also represents the energy flux density. For scalar fields, the momentum density can be written as a local expectation value of the canonical momentum operator , where ψ ( r ) is the wave function, and we use units ħ =1. However, for vector fields, an additional spin momentum density was introduced in 1939 by F.J. Belinfante [27] to explain the spin of quantum particles and symmetrize the canonical energy-momentum tensor in field theory. The spin momentum is added to the canonical (or orbital) momentum density, resulting in [26] , [27] , [28] , [29] , [30] , [31] : Here is the spinor wave function, whereas s ( r ) is the spin AM density defined as the local expectation value of the corresponding matrix spin operator Ŝ : Equations (3) and (4) are fundamental and hold true for various particles. For Dirac electron, Ŝ is the spin-1/2 operator and is the Dirac bi-spinor [28] , [29] , [30] , [31] . In the case of monochromatic electromagnetic waves (photons), equation (3) yields the time-averaged Poynting vector p = γ k Re( E * × H ), when Ŝ is given by spin-1 matrices that act on the complex electric and magnetic field amplitudes, , supplied with the free-space Maxwell equations [22] , [26] , [27] , [28] , [29] , [30] , [31] (see Supplementary Note 1 ). Explicitly, the optical momentum and spin densities (3) and (4) read Note that these quantities are naturally split into electric and magnetic field contributions: and s = s e + s m . It is important to emphasize that although the Poynting vector p is usually considered in optics as a single momentum density of light [2] , it actually represents the sum of two quantities p O and p S , with drastically different physical meanings and properties. Below we uncover the contrasting manifestations of the canonical and spin momenta. The canonical (orbital) and spin parts of the momentum density (3), p = p O + p S , generate, respectively, the orbital and spin parts of the AM density: j=l+s (refs 26 , 27 , 32 , 33 ). The orbital AM density is l = r × p O , and this is an extrinsic origin-dependent quantity. At the same time, the spin AM density s , equation (4), is intrinsic (origin-independent). Nonetheless, its integral value is determined by the circulation of the spin momentum: S =∫ s dV =∫ r × p S dV , where integration by parts should be performed [28] , [29] , [30] , [31] , [32] , [33] . The orbital momentum density p O is naturally proportional to the local phase gradient (wave vector) in the field [22] . In contrast, Belinfante’s spin momentum p S is a rather enigmatic quantity [26] , [27] , [28] , [29] , [30] , [31] , [32] , [33] . On the one hand, the spin momentum provides the physical origin of the spin AM of quantum particles. On the other hand, it is usually considered as an auxiliary ‘virtual’ quantity, which cannot be observed per se . Indeed, the spin momentum represents a solenoidal current, which does not contribute to the energy transport ( ∇ ·p S =0 and ∫ p S dV =0), and only generates spin AM. Consider, for instance, the elliptically polarized electromagnetic plane wave (1). This field carries only the longitudinal orbital momentum density: , while the spin momentum vanishes: p S =0. In this case, what generates the spin AM density ? This known paradox [26] , [34] , [35] is resolved by representing the zero transverse momentum as an array of infinitely small loops of circulating spin momentum in the ( x,y ) plane [26] , [30] , [31] , [32] , see Fig. 1b . Currents from the neighbouring loops cancel each other, but at the same time they provide non-zero circulation along any finite closed loop, that is, non-zero spin AM along the z axis. The formal integral relation between p S and s does not work here, because a plane wave is an unbounded state; the introduction of a boundary (for example, Gaussian intensity distribution in the transverse plane) immediately produces a non-zero boundary spin current p S ≠0 with the integral circulation yielding the spin S (refs 28 , 30 , 31 , 32 ). Thus, Belinfante’s spin momentum is similar to the boundary magnetization current or topological quantum-Hall current in solid-state systems (multiple current loops are produced there by electron orbitals), whereas the spin AM is analogous to the bulk magnetization in such systems. Probing the momentum and spin densities with small particles Having the above theoretical picture, let us consider measurements of the momentum and spin densities in an electromagnetic field. As we mentioned in the Introduction, a small absorbing particle immersed in the field can be employed as a natural meter of these quantities. Calculating the radiation force and torque on a dipole Rayleigh particle with equal electric and magnetic polarizabilities, α e =α m =α, one can show that they are determined by the canonical momentum and spin densities [19] , [20] , [21] , [22] , [23] , [24] , [25] (see Supplementary Note 3 ): Here is the energy density of the field. The first term in the first equation (6) is the gradient force, while the second term is the radiation pressure force. Together they ‘measure’ the imaginary and real parts of the complex canonical momentum: , which is proportional to the quantum weak value of the photon’s momentum, (refs 19 , 22 , 36 ). Importantly, it is the canonical momentum p O rather than the Poynting vector p that represents the physicallymeaningful momentum density of light that appears in experiments ( p = p O only in linearly polarized paraxial fields and plane waves) [19] , [33] . In particular, the orbital and spinning motions of probe particles in circularly-polarized vortex beams [15] , [16] , [17] , [18] originate exactly due to the force from the azimuthal component of p O and the torque from the longitudinal component of the spin density s . Furthermore, the quantum-mechanical resonant momentum transfer from light to a two-level atom is also determined by the canonical momentum density [37] , [38] . Finally, a remarkable recent experiment [36] , which realized quantum weak measurements of the local momentum of photons, also measured p O (ref. 19 ). Thus, the spin momentum p S turns out to be indeed ‘virtual’, that is, non-observable for weak-interaction measurements. Note that we considered an ‘ideal’ particle with equal electric and magnetic polarizabilities. In reality, local light–matter interactions usually have electric character, and |α e |>>|α m |. This is because of the fundamental electric–magnetic (dual) asymmetry of matter, which breaks the intrinsic dual symmetry of the free space Maxwell equations [33] , [39] , [40] . In this case, the particle will ‘measure’ only the electric parts of the momentum and spin densities (5): and T ≃ γ −1 Im(α e ) s e (refs 25 , 33 ) (see Supplementary Note 3 ). The electric and magnetic contributions to the local dynamical characteristics of light are equivalent in paraxial propagating fields [22] : , s e ≃ s m , but they can differ significantly in other cases. Extraordinary momentum and spin in a single evanescent wave We are now in a position to consider the main subject of the present study: evanescent waves. A single evanescent wave propagating along the z axis and decaying in the x >0 half-space can formally be obtained via a rotation of the propagating plane wave (1) by an imaginary angle about the y axis [41] . In doing so, we obtain the electric evanescent-wave field: Here is the longitudinal wave number, whereas is the exponential decay rate, so that the complex wave vector is . Substituting field (7), with the corresponding magnetic wave field (see Supplementary Note 2 and Supplementary Fig. 2 ), into equations (3) and (5), we calculate the canonical momentum, spin momentum and spin AM densities in the evanescent wave: where w = γω | A | 2 exp(−2 κx ) is the spatially-inhomogeneous energy density of the wave. Equations (8) and (9) reveal remarkable peculiarities of the momentum and spin in evanescent waves and represent the key analytical point of our study. First, note that the evanescent wave (7) possesses longitudinal canonical momentum , which exceeds the momentum of a plane wave with the same local intensity. Divided by the energy density w , this momentum yields the superluminal local group velocity in evanescent waves: v g z = ck z / k > c (refs 19 , 42 ). Although the Poynting vector corresponds to subluminal propagation, , it is the canonical momentum that represents the observable momentum density. In particular, the momentum transfer via the radiation force (6) to a dipole particle in the evanescent wave (7) will be larger than k per photon [43] . Such ‘super-momentum’ transfer was observed by Huard and Imbert [37] in the resonant Doppler coupling with a moving atom. In terms of the quantum weak measurements paradigm, the ‘super momentum’ represents a weak value of the photon momentum with the post selection in a ‘forbidden’ zone unreachable for propagating waves (for example, beyond a totally reflecting interface) [19] . However, what is much more intriguing in equations (8) and (9) is the presence of the transverse y -components of the momentum and spin in the wave (7) propagating solely within the ( x,z ) plane. Moreover, here the momentum becomes proportional to the helicity σ , while the spin s y ∝ ( κ / k z ) w turns out to be helicity independent! This is in sharp contrast to propagating waves and photons, equation (2). The transverse momentum and spin appear due to the two features of the evanescent field (7). The first one is the imaginary longitudinal component of the field polarization: . This induces a rotation of the fields in the propagation ( x,z ) plane (see Fig. 2a,d ), and generates the spin independently of σ . Recently, we described such spin for surface plasmon-polaritons [42] , and it was shown that the imaginary longitudinal field component plays an important role in optical coupling processes [44] , [45] . The second feature is the inhomogeneous intensity w ∝ exp(−2 κ x ). This inhomogeneity destroys the cancellation of the spin momentum loops in the ( x,y ) plane, which results in the non-zero transverse Belinfante’s spin momentum: , see Fig. 2e . Note that although equation (8) and Fig. 2b,e show unidirectional spin momentum in the x >0 half-space, the accurate consideration of the interface x =0 and medium in the x <0 half-space ensures the vanishing of the integral spin momentum, in agreement with ∫ p S dV =0 (ref. 42 ). 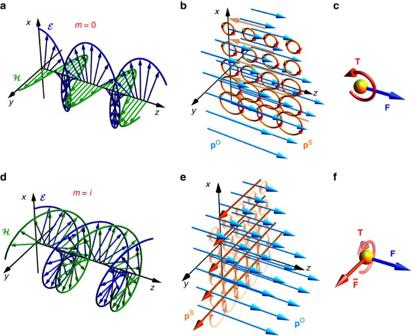Figure 2: Momentum and spin in linearly and circularly polarized evanescent plane waves. The complex wave electric field is given by equation (7) withm=σ=0 for the linear-polarization case (a–c) andm=i,σ=1 for the circular-polarization case (d–f). (a,d) The imaginary longitudinal components of the complexE(r) andH(r) fields (7) result in a cycloid-like projection of the instantaneous electric and magnetic field distributions, (r,t) and (r,t), onto the propagation (x,z) plane (seeSupplementary Note 2andSupplementary Fig. 2). As the wave propagates, the fields rotate in this plane even at linear polarizations. This rotation generates a transverse helicity-independent spin AM (8)sy∝(κ/kz)w, represented in (b) by multiple loops of the spin momentumpSin the (x,z) plane. Due to the vertical inhomogeneityw(x), these loops do not cancel each other, producing a backward spin momentum(semitransparent arrows). The circularly-polarized evanescent wave (d) also carries the usual longitudinal spinsz∝σwshown in (e) by multiple semitransparent loops of the spin momentum in the (x,y) plane (cf.Fig. 1). Due to the vertical inhomogeneityw(x), these loops produce transverse helicity-dependent spin momentum (8). The evanescent wave also possesses polarization-independent ‘superluminal’ orbital momentum (8). (c,f) The orbital momentum and spin AM are locally transferred to the probe particle thereby exerting: an anomalously large radiation force; the usual longitudinal helicity-dependent torqueTz∝sz; and the transverse helicity-independent torqueTy∝sy, equation (6). The transverse spin momentumdoes not exert radiation pressure in the dipole approximation (6), but does produce a helicity-dependent transverse force (10)(f) in higher-order interactions with larger Mie particles (seeFig. 3). Figure 2: Momentum and spin in linearly and circularly polarized evanescent plane waves. The complex wave electric field is given by equation (7) with m = σ =0 for the linear-polarization case ( a – c ) and m = i , σ =1 for the circular-polarization case ( d – f ). ( a , d ) The imaginary longitudinal components of the complex E ( r ) and H ( r ) fields (7) result in a cycloid-like projection of the instantaneous electric and magnetic field distributions, ( r , t ) and ( r , t ), onto the propagation ( x , z ) plane (see Supplementary Note 2 and Supplementary Fig. 2 ). As the wave propagates, the fields rotate in this plane even at linear polarizations. This rotation generates a transverse helicity-independent spin AM (8) s y ∝ ( κ / k z ) w , represented in ( b ) by multiple loops of the spin momentum p S in the ( x , z ) plane. Due to the vertical inhomogeneity w ( x ), these loops do not cancel each other, producing a backward spin momentum (semitransparent arrows). The circularly-polarized evanescent wave ( d ) also carries the usual longitudinal spin s z ∝ σ w shown in ( e ) by multiple semitransparent loops of the spin momentum in the ( x , y ) plane (cf. Fig. 1 ). Due to the vertical inhomogeneity w ( x ), these loops produce transverse helicity-dependent spin momentum (8) . The evanescent wave also possesses polarization-independent ‘superluminal’ orbital momentum (8) . ( c , f ) The orbital momentum and spin AM are locally transferred to the probe particle thereby exerting: an anomalously large radiation force ; the usual longitudinal helicity-dependent torque T z ∝ s z ; and the transverse helicity-independent torque T y ∝ s y , equation (6). The transverse spin momentum does not exert radiation pressure in the dipole approximation (6), but does produce a helicity-dependent transverse force (10) ( f ) in higher-order interactions with larger Mie particles (see Fig. 3 ). Full size image Relation to the Fedorov-Imbert controversy Here we should make a historical digression and note that an example of the transverse helicity-dependent momentum in an evanescent field was first found by F.I. Fedorov in 1955 (ref. 46 ). Incidentally, this discovery caused a half-century-long controversy in the physics of light reflection and refraction. Analysing the total internal reflection of a polarized plane wave, Fedorov found a helicity-dependent transverse component of the Poynting vector in the transmitted evanescent field. Fedorov concluded that ‘the lateral energy flux should lead to a specific light pressure’ and (by an analogy with the Goos–Hänchen effect) that ‘the reflected beam in the case of total reflection must be displaced in the lateral direction’. Later, C. Imbert indeed observed such helicity-dependent beam shift experimentally [47] , and the effect is now known as the Imbert–Fedorov transverse shift or spin Hall effect of light (for a review, see ref. 48 ). The 50 years after Fedorov’s finding brought about numerous controversies about this effect. Finally, only recently an accurate theoretical description was given [49] , [50] , which was followed by a precise experiment [51] using quantum weak measurements (see also refs 52 , 53 ). Remarkably, the current theory of the spin Hall effect of light is completely unrelated to evanescent waves and their transverse momentum. Indeed, the helicity-dependent beam shift arises from the interference of multiple plane waves in the beam, taking into account the geometric-phase effect, that is, the spin-orbit interaction of light [48] . This shift occurs in partial reflection or refraction, focusing, scattering and other optical phenomena without any evanescent waves. Thus, curiously, Fedorov predicted two fundamental helicity-dependent but unrelated phenomena (transverse momentum and beam shift) using a fictitious connection between them. Now, from equations (3) and (8), we can conclude that Fedorov’s transverse momentum is an example of Belinfante’s spin momentum, which does not transport energy and therefore cannot shift the field. Interaction of the evanescent wave with Mie particles The evanescent field (7) represents an exceptional configuration with a pure spin momentum without any orbital part in the transverse y -direction. This offers a unique opportunity to investigate this fundamental field-theory quantity per se . Equation (6) show that the spin momentum does not appear in the dipole interaction with small point-like particles. But does this result hold true for larger particles and higher-order interactions? To address this question, we examine the interaction of the evanescent optical field with finite-size Mie particles. The Mie scattering theory provides an exact solution for the plane-wave interaction with an isotropic spherical particle. Using the Maxwell stress tensor, one can calculate the flux of the momentum and AM through a sphere enclosing the particle, and thereby determine the force and torque acting on the particle [54] . Recently, we developed and successfully tested an extension of the Mie theory (based on complex-angle rotation of the standard theory), which describes the scattering of the incident evanescent wave (7) [41] (see also refs 55 , 56 ). Using this exact semi-analytical method, we calculate the radiation force and torque acting on the particle of radius a , complex permittivity ε p , and permeability μ p , immersed in the evanescent field (7). 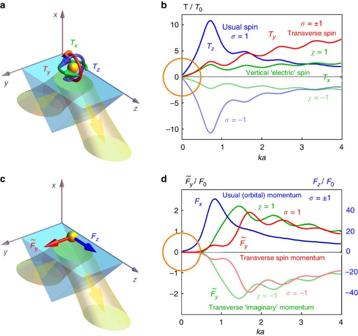Figure 3: Numerically calculated forces and torques on a Mie particle in an evanescent field. (a,c) Schematics of a proposed experiment (see alsoSupplementary Fig. 3). A polarized propagating wave undergoes total internal reflection at the glass–water interface, thereby generating the evanescent wave (7) in water. A gold spherical particle of radiusais placed in water on the glass surface, and its observable linear and spinning motion is proportional to the forces and torques exerted by the evanescent wave. (b,d) Normalized torque and force components for circular (m=±i,σ=±1) and diagonal (m=χ=±1) polarizations versus the particle sizeka(the Rayleigh dipole regionka≪1 is indicated by the orange circles). (b) The longitudinal helicity-dependent torqueTz∝sz∝σindicates the usual spin. The transverse torque is helicity independent and signals the appearance of the transverse spin (9):Ty∝sy∝(κ/kz)w. The vertical torque for the diagonal polarizationsχ=±1 appears because of the strong electric–magnetic (dual) asymmetry of the particle. It is caused by the non-zero electric part (10) of the (zero-net) vertical spin density:,sex=−smx. (d) The orbital momentum density (8) produces mostly polarization-independent longitudinal radiation pressure force:. At the same time, the transverse forcevanishes in the Rayleigh region, but becomes non-zero for larger Mie particles withka~1, see equation (11). This transverse force has the helicity-dependent part proportional to the transverse spin momentum (8):, and also theχ-dependent part proportional to the ‘imaginary’ Poynting momentum (12). Figure 3a,c shows the schematic of the corresponding experiment using the total internal reflection at a glass prism. For this numerical experiment, we use parameters corresponding to real experiments manipulating particles with evanescent fields (for example see refs 57 , 58 , 59 , 60 , 61 , 62 ). Namely, we consider radiation with the wavelength λ =650 nm, a gold particle ( ε p =−12.2+3 i , μ p =1) in water ( ε =1.77, μ =1), and near-critical total internal reflection (the angle of incidence is θ =51°= θ c +1.5°) from the interface between heavy flint glass ( ε 1 =3.06, μ 1 =1) and water. Calculations of the corresponding wave fields and characteristics are given in the Supplementary Notes 2 and 3 . The resulting force and torque components (normalized by F 0 = a 2 | A 1 |/4 π and T 0 = F 0 / k , with A 1 being the amplitude of the incident wave in the glass), as functions of the dimensionless particle radius ka are shown in Fig. 3b,d (see also Supplementary Fig. 4 and Supplementary Table 1 ). These are the main numerical results of our work, which offer several new experiments for the detection of extraordinary spin and momentum properties of evanescent waves. Figure 3: Numerically calculated forces and torques on a Mie particle in an evanescent field. ( a , c ) Schematics of a proposed experiment (see also Supplementary Fig. 3 ). A polarized propagating wave undergoes total internal reflection at the glass–water interface, thereby generating the evanescent wave (7) in water. A gold spherical particle of radius a is placed in water on the glass surface, and its observable linear and spinning motion is proportional to the forces and torques exerted by the evanescent wave. ( b , d ) Normalized torque and force components for circular ( m =± i , σ =±1) and diagonal ( m = χ =±1) polarizations versus the particle size ka (the Rayleigh dipole region ka ≪ 1 is indicated by the orange circles). ( b ) The longitudinal helicity-dependent torque T z ∝ s z ∝ σ indicates the usual spin. The transverse torque is helicity independent and signals the appearance of the transverse spin (9): T y ∝ s y ∝ ( κ / k z ) w . The vertical torque for the diagonal polarizations χ =±1 appears because of the strong electric–magnetic (dual) asymmetry of the particle. It is caused by the non-zero electric part (10) of the (zero-net) vertical spin density: , s e x =− s m x . ( d ) The orbital momentum density (8) produces mostly polarization-independent longitudinal radiation pressure force: . At the same time, the transverse force vanishes in the Rayleigh region, but becomes non-zero for larger Mie particles with ka ~1, see equation (11). This transverse force has the helicity-dependent part proportional to the transverse spin momentum (8): , and also the χ -dependent part proportional to the ‘imaginary’ Poynting momentum (12) . Full size image Figure 3b depicts the radiation torque components for right-hand and left-hand circularly-polarized waves ( m =± i , σ =±1). While the longitudinal torque T z from the usual spin s z flips with the sign of σ , the transverse torque T y is helicity-independent and present even in the linear-polarization Im m =0 case. This confirms the presence of the transverse helicity-independent spin AM (8) s y in the evanescent field and its transfer to the particle. For small Rayleigh particles, ka <<1, the torque is described by the dipole approximation (6). Due to the strong dual (electric–magnetic) asymmetry of the gold, the torque appears mostly from the electric part of the spin (5): T ≃ γ −1 Im(α e ) s e , where the electric polarizability is proportional to the particle’s volume: α e ∝ ( ka ) 3 , while the magnetic polarizability is small: α m ∝ ( ka ) 5 ≃ 0 (refs 63 , 64 ). Therefore, the transverse torque is maximal for the TM-mode with m =0 and s y = s e y , and minimal for the TE-mode with m =∞ and s y = s m y (see Supplementary Notes 2 and 3 ). The dual asymmetry results in another remarkable effect. Namely, for waves linearly diagonally-polarized at ±45° ( m =±1), a vertical radiation torque T x appears, which is proportional to the degree of diagonal polarization . This torque signals the presence of the vertical electric spin component: which arises from the diagonal-electric-field rotation in the ( y , z )-plane (see equation (7) and Supplementary Note 2 ). Importantly, the total vertical spin vanishes in (9), because the electric and magnetic fields rotate in opposite directions: s x = s e x + s m x =0. Nonetheless, the dual-asymmetric gold particle unveils the electric vertical spin (10), as shown in Fig. 3b . Figure 3d shows the longitudinal and transverse components of the radiation force for circular ( m =± i , σ =±1) and diagonal ( m = χ =±1) polarizations. The longitudinal force F z represents the radiation pressure (mostly polarization-independent) from the orbital momentum . Akin to the torque, it exhibits an effective electric-dipole interaction in the Rayleigh regime ka <<1. The transverse force vanishes in this regime, F y =0, which confirms the ‘virtual’ character of the spin momentum. Nonetheless, a non-zero helicity-dependent transverse force arises for larger Mie particles with ka ~1. This force originates from the higher-order interaction between electric- and magnetic-induced dipoles, and in the quadratic dipole–dipole approximation it can be written as [63] , [64] (see Supplementary Note 3 ) Here we introduced the complex Poynting momentum: , with being the usual Poynting vector and characterizing an alternating flow of the so-called ‘stored energy’ [2] . Alongside with the transverse σ -dependent spin momentum (8) , the evanescent wave (7) possesses a χ -dependent transverse imaginary Poynting momentum (see Supplementary Note 3 ) These two transverse momenta determine two contributions to the transverse dipole–dipole force (11): . In complete agreement with this, numerical calculations in Fig. 3d show σ -dependent and χ -dependent transverse radiation forces on Mie particles with ka ~1, which vanish as ∝ α e α m ∝ ( ka ) 8 at ka <<1. This proves the presence and observability of the transverse Belinfante’s spin momentum in the evanescent optical field. Detailed analysis and calculations of all torque and force components for all basic polarizations m =0,∞,± i ,±1 can be found in the Supplementary Note 3 , Supplementary Figs 4 and 5 , and Supplementary Table 1 . To summarize, we have found that a single evanescent electromagnetic wave offers a rich and highly non-trivial structure of the local momentum and spin distributions. In sharp contrast to standard photon properties, evanescent waves carry helicity-independent transverse spin and helicity-dependent transverse momentum. Moreover, the transverse momentum turns out to be a fundamental spin momentum introduced by Belinfante in field theory and first remarked in optics (as an unusual Poynting vector) by Fedorov. We have examined the measurements of the extraordinary spin and momentum in the evanescent field by analysing its interaction with a probe particle. Analytical evaluations and exact numerical simulations based on parameters of typical optical-manipulation experiments show that the transverse helicity-independent spin (and also the vertical electric spin for diagonal polarizations) can be detected straightforwardly via the radiation torque exerted on an absorbing small particle. At the same time, the Belinfante–Fedorov’s spin momentum does not exert the standard optical pressure in the dipole approximation, which confirms its ‘virtual’ character (in contrast to Fedorov’s interpretation). Nonetheless, it appears detectable (in contrast to the field-theory interpretation) via a helicity-dependent transverse optical force from the higher-order interaction with Mie particles. Thus, an exceptional evanescent- wave structure with pure spin transverse momentum offers a unique opportunity for the direct observation of this fundamental field-theory quantity, which was previously considered as ‘virtual’. In total, this work offers four novel experiments for the detection of extraordinary momentum and spin properties of a single evanescent wave (red and green curves in Fig. 3 ). These proposed experiments could detect the following optical torques and forces. First, the transverse helicity-independent torque T y indicating the transverse spin s y ( Fig. 3b , equations (6) and (9)). Second, the vertical diagonal-polarization-dependent torque T x exerted on a dual-asymmetric (for example, electric-dipole) particle and caused by the vertical electric spin s e x ( Fig. 3b and equation (10)). Third, the transverse helicity-dependent force produced by the transverse spin momentum ( Fig. 3d , equations (8) and (11)). Fourth, the transverse diagonal-polarization-dependent force , which is associated with the transverse imaginary Poynting vector ( Fig. 3d , equations (11) and (12)). These results add a distinct chapter in the physics of momentum and spin of classical and quantum fields, and offers a variety of non-trivial light-matter interaction effects involving evanescent fields. How to cite this article: Bliokh, K. Y. et al. Extraordinary momentum and spin in evanescent waves. Nat. Commun. 5:3300 doi: 10.1038/ncomms4300 (2014).